Practice and sleep form different aspects of skill Performance for skills such as a sequence of finger movements improves during sleep. This has widely been interpreted as evidence for a role of sleep in strengthening skill learning. Here we propose a different interpretation. We propose that practice and sleep form different aspects of skill. To show this, we train 80 subjects on a sequence of key-presses and test at different time points to determine the amount of skill stored in transition (that is, pressing ‘2’ after ‘3’ in ‘4-3-2-1’) and ordinal (that is, pressing ‘2’ in the third ordinal position in ‘4-3-2-1’) forms. We find transition representations improve with practice and ordinal representations improve during sleep. Further, whether subjects can verbalize the trained sequence affects the formation of ordinal but not transition representations. Verbal knowledge itself does not increase over sleep. Thus, sleep encodes different representations of memory than practice, and may mediate conversion of memories between declarative and procedural forms. The now well-established and accepted case for a role of sleep in strengthening or enhancing a procedural skill has largely been built upon findings that finger sequencing skill improves with both practice and over a period of sleep [1] , [2] . Further, it is known that sequencing requires the formation of memory representations for certain types of information contained inherent in sequences such as movement to movement transitions, and ordinal positions of movements within a sequence [3] , [4] , [5] , [6] , [7] , [8] , [9] . Dissociations in learning for transition and ordinal information in humans, chimpanzees, monkeys and pigeons have been demonstrated [5] , [9] , suggestive of a neurobiological distinction. Learning of transitions is present in humans (who can learn transition probabilities from up to six items prior [6] ) and monkeys (who can learn transitions between consecutive items [5] , [9] ), but not in pigeons [9] . On the other hand, learning the ordinal position of events in four-item lists has been demonstrated in humans [8] , monkeys [3] and pigeons [7] . In a real-life setting, for an experienced pianist, familiarity with frequencies of movement-to-movement transitions within a musical key can lead to faster performance of a new song that is written in a key rather than out of key, while each new song within a key can be unique, with this uniqueness represented by the ordinal position of each of the movements. Motor skills for hobbies such as these and for compulsory activities such as speaking and driving, rely in part on the human ability to form long-term memory representations of both transition and ordinal information [4] , [5] , [6] , [8] , [9] . Though it is known that a period of practice improves skill (online gains) as does a period of sleep (offline overnight gains) [1] , [10] , it is not known whether online and overnight gains encode the same type of information. Here we show online gains develop for transition information and overnight gains for ordinal information. Further, ability to verbalize a sequence affects the overnight formation of ordinal representations only. Thus, practice and sleep contribute to different aspects of skill. Study design to assess stages of motor learning Eighty subjects were trained on a repeating 12-item sequence of key-presses ( Fig. 1a ) and performance of the same sequence of key-presses was tested at various time points: before training (baseline), 5 min after training (end), and at 12h, 24 h and 1 week after training ( Fig. 1b , see Methods). With this design, online gains could be determined by baseline and end of training comparisons, while overnight and over-day gains could be assessed by comparing end of training and subsequent 12-h delays. Long-term retention of gains was tested 1 week after training. 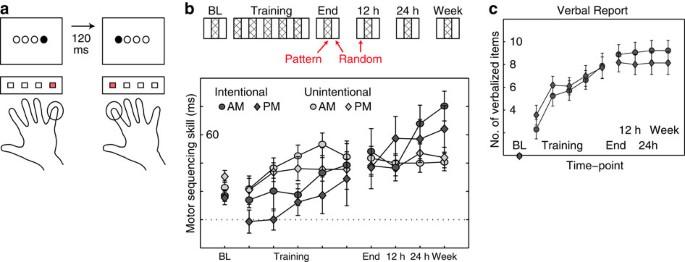Figure 1: Study design assesses stages of motor learning. (a) Eighty subjects made a key-press response with one of four fingers of the right hand in response to a visuo-spatial target appearing in one of four locations on a computer screen (see Methods). (b) In random blocks (empty), targets were randomly ordered throughout the block. In pattern blocks (hatched), targets followed a 12-item sequence (repeated eight times). Subjects’ performance was tested on a pattern block at five time points: baseline (BL), 5 min after training (end), after 12 h, after 24 h and after 1 week. Five pattern blocks were practiced during training. Two random blocks flanked each pattern block during test times, and training also included five random blocks interspersed. Motor sequencing skill was assessed as the difference in response times between random and pattern blocks (raw scores inSupplementary Fig. 1C). A 10 × 2 × 2 ANOVAMD(time point × instruction × AM/PM) revealed a main effect of time point:n=79, F1,4.3=10.0,P<0.0001, and a time point by instruction interaction: F1,4.3=3.5,P<0.008. Error bars are s.e.m. (c) In intentional learners, the number of items belonging to any of the verbalized trains was plotted and a 10 × 2 ANOVAMD(time point × AM/PM) revealed a main effect of time point:n=39, F1, 5.2=36.6,P<0.0001. Error bars are s.e.m. Figure 1: Study design assesses stages of motor learning. ( a ) Eighty subjects made a key-press response with one of four fingers of the right hand in response to a visuo-spatial target appearing in one of four locations on a computer screen (see Methods). ( b ) In random blocks (empty), targets were randomly ordered throughout the block. In pattern blocks (hatched), targets followed a 12-item sequence (repeated eight times). Subjects’ performance was tested on a pattern block at five time points: baseline (BL), 5 min after training (end), after 12 h, after 24 h and after 1 week. Five pattern blocks were practiced during training. Two random blocks flanked each pattern block during test times, and training also included five random blocks interspersed. Motor sequencing skill was assessed as the difference in response times between random and pattern blocks (raw scores in Supplementary Fig. 1C ). A 10 × 2 × 2 ANOVA MD (time point × instruction × AM/PM) revealed a main effect of time point: n =79, F 1,4.3 =10.0, P <0.0001, and a time point by instruction interaction: F 1,4.3 =3.5, P <0.008. Error bars are s.e.m. ( c ) In intentional learners, the number of items belonging to any of the verbalized trains was plotted and a 10 × 2 ANOVA MD (time point × AM/PM) revealed a main effect of time point: n =39, F 1, 5.2 =36.6, P <0.0001. Error bars are s.e.m. Full size image After baseline half of the subjects were told there was a repeating 12-item sequence that they would be asked to verbally report after each pattern block (intentional group) while the other half was not told (unintentional group). To control for the influence of circadian factors on performance measures, we trained subjects in each group either early in the morning (between 07:00 and 09:00 h, AM groups) or later at night before sleep (between 19:00 and 21:00 h, PM groups). Thus, there were a total of four groups (intentional-AM, intentional-PM, unintentional-AM and unintentional-PM). Motor sequencing skill at each time point was assessed by comparing response times in pattern blocks, where trials followed the repeating 12-item sequence, and in random blocks, where trials were randomly ordered [11] ; Fig. 1b ). Motor sequencing skill was influenced by the instructions subjects received (10 × 2 × 2 ANOVA MD main effect of time point: n =79, F 1,4.3 =10.0, P <0.0001), and time point by instruction interaction: F 1,4.3 =3.5, P <0.008. It is possible that the time point by instruction interaction was driven by the initial slowing during training blocks with declarative learning in intentional learners [12] . Raw response time and accuracy scores are displayed in Supplementary Fig. 1C . Accuracy for both groups remained high averaging 96±2% across the entirety of the study. In intentional learners, the number of verbalized items increased, indicating increasing ability to verbalize the sequence (10 × 2 ANOVA MD main effect of time point: n =39, F 1, 5.2 =36.6, P <0.0001, Fig. 1c ). Skill at each time point was parsed into transition and ordinal-based representations by first mathematically modelling the influence of conditional probabilities of transitioning on response time to calculate transition-based representations (principle component regression, see Methods, Supplementary Fig. 2A and Supplementary Fig. 2C ) and second by comparing response times between short identical trains of trials in random and pattern blocks while removing contributions of higher-order differences in transitioning for ordinal-based representations (see Methods and Supplementary Fig. 2B ). Practice encodes transition-based representations With practice, overall motor sequencing skill improved online (2 × 2 ANOVA MD : n =79, F 1,77 =8.9, P <0.004). However, while transition-based representations improved substantially (2 × 2 ANOVA MD : n =79, F 1,1 =56.8, P <0.0001), ordinal-based representations during practice did not ( Fig. 2a ). Online transition-based gains retained to 1 week ( Fig. 2e ). Further post hoc analyses on online transition-based gains assessing first to sixth orders of conditional probability (OC) of transitioning (first OC takes into account transition information from n -1, second OC additionally from n -2, third OC additionally from n -3 and so on) showed that transition representations relied on lower OCs (from second) more than higher OCs ( Fig. 2a bottom, 2 × 2 × 6 ANOVA MD main effect of OC: n =79, F 1,2.8 =34.9, P <0.0001 and OC by online interaction: F 1,3.0 =12.2, P <0.0001). 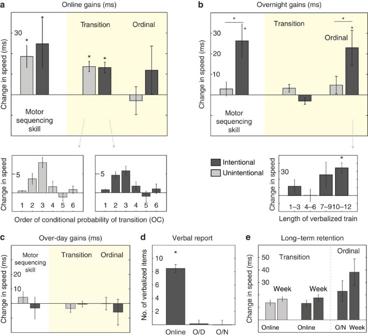Figure 2: Practice encodes transition-based representations and sleep encodes ordinal-based representations of a skill memory. (a) Online gains: motor sequencing skill improved online (2 × 2 ANOVAMD(online × instruction) main effect of online:n=79, F1,77=8.9,P<0.004) in both groups (t-tests: unintentionaln=40, t(39)=3.4,P<0.002, intentional:n=39, t38=2.1,P<0.05, Bonferroni corrected). Online improvements were only evident for transition-based information (2 × 2 ANOVAMD:n=79, F1,1=56.8,P<0.0001) and in both groups (t-tests: unintentionaln=40, t39=5.6,P<0.0001, intentionaln=39, t38=5.1,P<0.0001, Bonferroni corrected). A 2 × 2 × 6 ANOVAMDassessing the contribution of first to sixth OC of transitioning on online gains revealed a main effect of OC:n=79, F1,2.8=34.9,P<0.0001 and an OC by online interaction: F1,3.0=12.2,P<0.0001. Ranking according to effect size (unintentional: third, second, fourth, sixth, first, fifth; intentional: third, second, fourth, sixth, first, fifth) suggest that lower OCs were learned faster than higher ones, with the exception of 1st OCs. Error bars are s.e.m. (b) Overnight gains: motor sequencing skill improved overnight but only in intentional learners (2 × 2 ANOVAMD(overnight × instruction) main effect of overnight:n=79, F1,77=7.5,P<0.008 and overnight by instruction interaction: F1,77=8.72,P<0.004;t-tests: intentionaln=39, t38=3.2,P<0.003, Bonferroni corrected). Overnight gains were only evident for ordinal-based information (2 × 2 ANOVAMDmain effect of overnight:n=79, F1,1=8.6,P<0.005 and overnight by instruction interaction: F1,77=3.8,P≤0.05;t-tests: intentional:n=39, t38=2.7,P<0.01, Bonferroni corrected).Post hoc t-tests revealed significant overnight ordinal-based gains only when trials belonging to long, 10–12-item verbalized trains (n=17, t16=3.1,P<0.03, Bonferroni corrected). Error bars are s.e.m. (c) No significant over-day gains in motor sequencing skill (nor representations) were detected. (d) In intentional learners, verbal knowledge was acquired online (pairedt-test,n=39, t38=14.1,P<0.0001) only. (e) To assess long-term retention, we compared significant online transition-based and significant overnight ordinal-based gains to long-term gains between 1 week and baseline and found no significant differences. Figure 2: Practice encodes transition-based representations and sleep encodes ordinal-based representations of a skill memory. ( a ) Online gains: motor sequencing skill improved online (2 × 2 ANOVA MD (online × instruction) main effect of online: n =79, F 1,77 =8.9, P <0.004) in both groups ( t -tests: unintentional n =40, t(39)=3.4, P <0.002, intentional: n =39, t 38 =2.1, P <0.05, Bonferroni corrected). Online improvements were only evident for transition-based information (2 × 2 ANOVA MD : n =79, F 1,1 =56.8, P <0.0001) and in both groups ( t -tests: unintentional n =40, t 39 =5.6, P <0.0001, intentional n =39, t 38 =5.1, P <0.0001, Bonferroni corrected). A 2 × 2 × 6 ANOVA MD assessing the contribution of first to sixth OC of transitioning on online gains revealed a main effect of OC: n =79, F 1,2.8 =34.9, P <0.0001 and an OC by online interaction: F 1,3.0 =12.2, P <0.0001. Ranking according to effect size (unintentional: third, second, fourth, sixth, first, fifth; intentional: third, second, fourth, sixth, first, fifth) suggest that lower OCs were learned faster than higher ones, with the exception of 1st OCs. Error bars are s.e.m. ( b ) Overnight gains: motor sequencing skill improved overnight but only in intentional learners (2 × 2 ANOVA MD (overnight × instruction) main effect of overnight: n =79, F 1,77 =7.5, P <0.008 and overnight by instruction interaction: F 1,77 =8.72, P <0.004; t -tests: intentional n =39, t 38 =3.2, P <0.003, Bonferroni corrected). Overnight gains were only evident for ordinal-based information (2 × 2 ANOVA MD main effect of overnight: n =79, F 1,1 =8.6, P <0.005 and overnight by instruction interaction: F 1,77 =3.8, P ≤0.05; t -tests: intentional: n =39, t 38 =2.7, P <0.01, Bonferroni corrected). Post hoc t -tests revealed significant overnight ordinal-based gains only when trials belonging to long, 10–12-item verbalized trains ( n =17, t 16 =3.1, P <0.03, Bonferroni corrected). Error bars are s.e.m. ( c ) No significant over-day gains in motor sequencing skill (nor representations) were detected. ( d ) In intentional learners, verbal knowledge was acquired online (paired t -test, n =39, t 38 =14.1, P <0.0001) only. ( e ) To assess long-term retention, we compared significant online transition-based and significant overnight ordinal-based gains to long-term gains between 1 week and baseline and found no significant differences. Full size image Sleep encodes ordinal-based representations Motor sequencing skill improved overnight (2 × 2 ANOVA MD main effect of overnight: n =79, F 1,77 =7.5, P <0.008 and overnight by instruction interaction: F 1,77 =8.72, P <0.004). However, while ordinal-based representations improved substantially (2 × 2 ANOVA MD main effect of overnight: n =79, F 1,77 =8.6, P <0.005 and an overnight by instruction interaction: F 1,77 =3.8, P ≤0.05), transition-based ones did not ( Fig. 2b ). Overnight ordinal-based gains retained to 1 week ( Fig. 2e ). Intention to learn the sequence significantly affected the appearance of overnight ordinal-based gains pointing to the possible importance of declarative knowledge of the sequence. This knowledge was assessed by verbal report, which showed significant gains ( Fig. 2d ). However, ordinal-based representations formed significantly only for trials that were part of long verbalized trains (10–12 in a row) that could be recounted prior to the overnight period ( Fig. 2b bottom, one-sample t -test: n =19, t 18 =3.1, P <0.04, Bonferroni corrected) and not for trials part of short verbalized trains (1–6 in a row, Fig. 2b bottom and Supplementary Table 2 ). Over-day gains were not detected pointing to sleep specificity rather than passage of time itself ( Fig. 2c ). Thus, our results show that practice can form skill based on transition information and sleep, ordinal information. Previous findings with motor sequencing tasks have suggested sleep consolidation functions to strengthen the motor memory encoded during practice but here for the first time, we demonstrate the formation of a different representation of a procedural skill during sleep. Sleep represents an oscillatory and neurochemically distinct state that can allow binding not possible during waking states [1] , [13] , [14] . Ordinal learning involves binding between an event and a spatio-temporal context, supported by the hippocampus [15] . During sleep, the hippocampus replays the sequence encountered earlier only at a condensed rate [16] , [17] and the unique brain state along with the condensed replay may support new encoding [1] , [18] , [19] . Similar to previous studies, we found greater sensitivity for lower (second and third) rather than higher (fourth and higher) OCs of transitions [6] , [20] with the exception of first OCs that are often ambiguous and hence, less predictive of future events [20] . Hence, transition information was encoded first online, and at a faster rate for lower order conditionals as would bind proximate events, while ordinal information was encoded overnight, and for long trains of verbalized trials as could bind together more distal events. This time course may provide a mechanism for long speculated theories on hierarchical processing for sequential information which propose two steps in learning, one for proximate events, and another for binding across the length of an entire sequence [5] . Practice encoded transition information to the same extent irrespective of whether or not the learner intended to learn the sequence. In contrast, sleep encoded ordinal information only when the subject intended to learn the sequence. Previous work has noted the necessity of intentional instruction, inclusive of ability to verbalize, for successful sleep-dependent enhancement of motor sequence learning [21] . This form of learning is related to sleep spindles [10] unlike that taking place under unintentional conditions, in which sleep specific changes are generally absent [11] , [21] , [22] , [23] or show complex interactions [24] , [25] . These complex interactions are proposed to occur between non-hippocampus-dependent and hippocampus-dependent memory systems, not only during performance but also during consolidation [25] . They may also occur between perception and movement-based coordinate frames [24] with studies showing transition information can be encoded in both coordinate frames [26] . These topics represent areas of future research. In the current study, we found a sleep effect only in trials that were clearly verbalized prior to the overnight period. Verbal knowledge showed online and not offline gains and hence, it is likely that one role of sleep is to translate declarative knowledge into procedural skill. Previous studies with amnesics such as H.M. indicate that in addition to procedural learning, older, consolidated declarative memories are not affected by lesions to the medial temporal lobes while newer declarative learning is impaired, a phenomenon known as the inverse-recency effect [27] . It is possible that sleep-dependent processes convert declarative memories into forms that behave more like procedural skills and this study may present one example of this. Attention is necessary for declarative learning and may represent the main determinant for whether or not sleep consolidates learning [28] . Studies have found that sleep can translate procedural into declarative knowledge [29] , [30] perhaps allowing for flexible encoding between its declarative and procedural forms [1] . Perhaps, the act of practicing in and of itself justifies encoding of transition information in procedural skill, while sleep needs additional resources to justify encoding of ordinal information that is goal-oriented and deemed important [28] . Malfunction of such a filter may link together sleep and diseased states such as schizophrenia where obscure associations and patterns take on inappropriate significance [31] . Though further study is necessary, it is clear that practice and sleep function to acquire different types of memory representation, allowing human beings to carry on a multitude of activities such as playing piano, conversing, driving and living through waking and sleeping. Subjects Eighty subjects gave their informed consent to the experimental procedure, which was approved by the National Institute of Neurological Disorders and Stroke (NINDS) Institutional Review Board (IRB) with minor deviations in the exact timings of the procedures that were reported to the IRB. One subject was excluded due to an error in data collection, for a total of 79 subjects (age, sex and neuropsychological characterization listed in Table 1 ). All subjects were right-handed and naive to the task and had a normal neurological examination as assessed by a credentialed physician. Sleep quality was assessed with the Pittsburg Sleep Questionnaire Inventory (PSQI) [32] and time of day preference with the Morningness-Eveningness Questionnaire (MEQ) [33] . Also, subjects were asked how many hours they had slept during the intervening overnight period between task delays (sleep and circadian characterization listed in Table 2 ). Eighty subjects were randomly assigned to one of four groups (intentional-AM, intentional-PM, unintentional-AM and unintentional-PM) with n =19 or 20 in each group. This group size is comparable to similar studies using the same task ( n =12 (ref. 25) [25] to n =25 (ref. 34) [34] per group). Table 1 Subject demographics and neuropsychological characterization. Full size table Table 2 Sleep and circadian factors characterization. Full size table Task and instructional manipulation Early work into sleep-dependent consolidation has often focused on intentional conditions and short finger tapping sequences of 5 or 9 items [2] , [35] , while later work has manipulated instruction (intentional and unintentional) and has employed 12-item sequences and the Serial Reaction Time Task (SRTT) [21] , which uses visual cues to guide finger movements. In this study, we used the SRTT and controlled differences in difficulty and construction/composition of the sequences [36] using a previously described method [11] , [34] : Specifically, a pattern sequence was randomly chosen for each subject from a corpus of 563 12-item sequences that contain no repetitions. For pattern blocks, this sequence was appended eight times in a row. For random blocks, eight different sequences were chosen at random without replacement from the corpus. There were no interruptions to mark the beginning of a new sequence (120 ms response to stimulus interval between items throughout the block). Between blocks, subjects saw a feedback screen of overall accuracy, which stayed onscreen for 30 s. After the feedback screen, subjects pressed any key to begin a new block. Instructions for the baseline blocks were identical across groups. Subjects were instructed to respond as fast as possible while aiming for perfect accuracy. Between baseline and the first training blocks, intentional subjects were asked if they had noticed a pattern (no subject reported that they had). They were then told that in half of the training blocks, the trials would follow a repeating sequence that was 12 items in length. The training instruction in this intentional group was to: ‘first and foremost, respond as fast as possible while aiming for perfect accuracy, second memorize the pattern, and lastly, if you noticed a pattern, tell me what it was, using the numbers 1–4 to represent the four key-presses’. Subjects in the unintentional group were not asked if they had noticed a pattern nor informed about the presence of a repeating sequence. They were solely instructed to: ‘respond as fast as possible while aiming for perfect accuracy’. Subjects in both groups were tested 5 min (end), 12 h, 24 h and 1 week after training. Immediately before each test, intentional subjects were informed about the location of the pattern block. After each test, they were again asked to verbally report back the pattern. Unintentional subjects on the other hand were told about the pattern at the end of the last test (1 week). At this time (end of 1 week testing), subjects in both groups were asked to recreate the repeating sequence using the process dissociation procedure (PDP [37] ). In intentional learners, verbal reports for pattern blocks were analysed as follows to avoid false positives. Since at least one correct pair can be recalled correctly by chance >99% of the time and at least one correct triplet >98% of the time, we chose to start with at least one correct quad which could be generated by chance 35% of the time. When a correct quad was reproduced, all four items were labelled correctly verbalized, and each subsequent correct item was added to this declarative train until the subject reported an incorrect item. If not even a correct quad was reproduced (or during the training period if the subject had not noticed the presence of a pattern in that block), the subject received a score of 1 for declarative knowledge in that block ( Fig. 1c ). This method was also used to identify the length of the verbalized train each item belonged to. Hence, items could be categorized either as non-verbalized (up to three in a row reported correctly), as belonging to a short verbalized train (four to six in a row reported correctly), a medium verbalized train (seven to nine in a row reported correctly) or a long verbalized train (10–12 in a row reported correctly) ( Fig. 2b bottom). At the end of the 1 week time point, both instructional groups completed motoric-free generation in accordance with the PDP, a sensitive measure of conscious recall [37] analysis detailed in ref 34 . In brief, subjects are asked to motorically regenerate the 12-unit pattern in inclusion blocks, and then avoid regenerating the pattern in exclusion blocks. Comparisons between the two blocks yield a measure of conscious recollection ( Supplementary Fig. 1A ). Analytic methods for task The amount of memory stored was derived in the following ways. First, total motor sequencing skill was calculated using the traditional method of comparing median response times between random and pattern blocks while keeping accuracy high through instruction [11] , [34] . For test blocks, comparisons were between the middle pattern block and flanking random blocks. For training, the first pattern block was compared with the first random block, the second pattern block to the second random block and so on. Means of medians were compared for group-wise statistical comparisons. Next, we calculated estimates for transition and ordinal-based representations of motor sequencing skill at each time point. Two methods for calculating these estimates are detailed in this section, including one employing principle component regression that mathematically models first to sixth order conditional probabilities of transition [6] , [20] , [38] , [39] and a second user-friendly subtractive method where triplet chunks containing high- and low-frequency transitions are identified and compared. Results from mathematical modelling are reported in the main text and results from the subtractive method are presented in Supplementary Fig. 3 . Key-press to key-press transitions in random blocks are random (excluding repetitions) and hence, on average, every transition occurs an equal number of times. However, due to the fact that some of these transitions are repeatedly practiced in pattern blocks, certain transitions in random blocks become higher frequency and others lower frequency, providing a large degree of variance in conditional probabilities of transitions in random blocks. Hence random blocks could be used to construct a model describing the relationship between variance in speed and variance in conditional probabilities of transitions, which could then be applied to pattern blocks to estimate transition-based representations. Specifically, for each subject, conditional probabilities of transition from the first to sixth order conditional (the X-terms) were calculated for every trial along the entire length of the task. If a trial such as 4 followed key-presses 13243 (as in …13243-4), then the first-order conditional probability of transition for that trial was calculated as the number of times ‘3-4’ appeared up until that trial divided by the number of times ‘3-n’ (‘3-1’, ‘3-2’, ‘3-4’) had appeared up until that trial. Second-order conditional probability of transition for that trial was calculated as the number of times ‘43-4’ appeared up until that trial divided by the number of times ‘43-n’ (‘43-2’, ‘43-1’, ‘43-4’) had appeared up until that trial. The third-order conditional probability of transition for that trial was calculated as the number of times ‘243-4’ appeared up until that trial divided by the number of times ‘243-n’ (‘243-1’, ‘243-3’, ‘243-4’) had appeared up until that trial (and so on and so forth). For each subject, for every random block, these X-terms were then demeaned and principle component analysis was applied to solve the issue of multi-collinearity between the conditional probabilities [39] (Matlab: princomp). The first three components were retained as together, they accounted for >85% of the total variance in the X-terms in every case (on average, the principal component analysis for each time point with first to sixth order conditional probabilities as input variables yielded a first factor explaining ~62% of total variance, a second factor explaining 18% and a third explaining 9%). Multiple linear regression was performed on the principal component matrix retaining these three orthonormal components and the demeaned response times at each trial (Matlab: lsqlin), and the regression coefficients for the components were then converted to regression coefficients for the original centred X-terms. Note that the X-terms were not scaled as the relative differences in variance were deemed potentially meaningful. Average variance in X-terms for each level of conditional probability is listed here: first: 0.017, second: 0.053, third: 0.087, fourth: 0.104, fifth: 0.106, sixth: 0.096. Once we derived this model describing the relationships between reaction time and conditional probabilities of transition for each subject for each random block at each time point, we could then apply this model to the pattern block at that time point, and derive an estimate for the transition-based representation of skill. For test blocks, we derived two models for the two random blocks flanking each pattern block, and averaged the regression coefficients to derive an average model to apply to the pattern block. The exception is baseline where only the second random block was used, as the initial block reflected familiarization with the task and inadequate variance in X-terms. For training blocks, the model for the first random block was used to calculate the transition-based representation of skill for the first pattern block, the model for the second random block was used to calculate the transition-based representation of skill for the second pattern block, and so on and so forth. In sum, we used conditional probabilities of transition in random blocks as X-terms and principle component regression to determine the relationship between variance in X-terms and variance in speed. Once we determined the regression coefficients, we had a model, wherein we could insert the average first through sixth order conditional probability of transition in the pattern block (as compared with the corresponding average in the random blocks) into the model and estimate the speed change that would occur based on conditional probability of transition. These estimates are reported in the main text. Another simple method for transition-based representations can be implemented without custom scripts. As stated, transitions in random blocks by chance bear semblance to transitions in pattern blocks and this method requires the identification of these trials that bear semblance, and trials that do not, and then simple subtraction of response times between the two. Specifically, each trial in the random blocks can be assigned to a triplet that includes the two preceding trials and if this triplet can be found in pattern blocks, this trial is labelled ‘pattern-like’. Otherwise, it is labelled ‘unlike’. Subtracting response times of ‘pattern-like’ and ‘unlike’ trials gives an estimate of transition-based representations. Intuitively this method makes sense, as one is isolating triplets in random blocks that share lower order transitions with pattern blocks to derive an estimate of transition representations. In addition, since these triplets are overlapping, they can also capture higher order transitions (‘4132’ contains ‘413’ and ‘132’ as pattern-like triplets). However, these estimates are predictably less accurate than the mathematical modelling method. The user-friendly method over-emphasizes lower order information. This is due to the fact that the mathematical method sets the average conditional probabilities for trials in a random block to the average response time for that random block, whereas in this user-friendly method, ‘pattern-like’ trials that are above the average conditional probabilities for lower orders are compared with ‘unlike’ trials that are below the average. Further, since triplets are employed, the user-friendly method under-estimates higher order contributions. Values derived from this user-friendly method are shown in Supplementary Fig. 3 . Key-press ‘3’ in ‘123214-3’ in a pattern block (in-place) shares the same transition information with a ‘3’ in ‘123214-3’ in a random block (out-place) but differences occur due to the presence of a set ordinal position in the pattern block. Hence, differences in speed between ‘in-place’ and ‘out-place’ trials would give estimates for ordinal-based representations. Practically, the number of times long trains occur in both pattern and random blocks are too sparse to directly compare. For example, there are 4 [7] possible combinations of seven-item trains given four possible key-press positions, although this would be lessened by lack of repeated key-presses from the task. For this reason, we focused on shorter ‘in-place’ and ‘out-place’ triplets and quadruplets, and then removed calculated contributions from higher order transitions (fourth and up for quadruplet-based analyses, third and up for triplet-based analyses). There is additional discussion relevant here on ‘absolute’ versus ‘relative’ ordinal position, as in: does ordinal position refer to being in the third ordinal position of the 12-unit sequence (relative) or being in the 47th ordinal position of the entire block (absolute)? Pragmatically, we could only look at relative ordinal learning due to the paucity of same and different ordinal positions of the absolute nature. At the same time, this allows us to conclude that ordinal-based representations observed in the current study is of the relative nature with virtually no contribution from absolute ordinal position information. As in transition-based measures, ordinal-based measures for test points were derived from comparisons between trials in the two flanking random blocks with the central pattern block, other than baseline where only the second random block was used, and for training blocks, where trials in the first random block were compared with trials in the first pattern block and trials in the second random block to the second pattern block and so on and so forth. For the subtractive method, comparisons of response times between ‘pattern-like’ trials in random blocks and response times of pattern trials give an estimate of ordinal representations. This estimate is less accurate as it does not take into account the differentials in higher order transition information. Values derived using this method are shown in Supplementary Fig. 3 . Statistical analyses To characterize a time course of learning, we employed mixed design ANOVAs with a within-subject factor of time course (baseline, train 1–5, end, 12 h, 24 h, week), and between-subject factors of instruction (intentional versus unintentional) and AM/PM (AM first or PM first). Prior to the ANOVA, sphericity was confirmed with Mauchly’s test. If the test for sphericity failed, we applied a Greenhouse–Geisser correction, which is reflected in the main text as a correction to the degrees of freedom. For our primary goal we wanted to confirm the absence or presence of online and offline gains (over-day and overnight) and we employed 2 × 2 mixed design ANOVAs with a within subjects factor of online/overnight/over-day (pre and post) and a between-subjects factor of instruction. Upon finding a significant effect of online (or overnight or over-day), we conducted post-hoc t -tests (one-tailed, with Bonferroni correction for multiple comparisons) to support statements that gains were evident. Unpaired t -tests were also employed to compare between groups (two-tailed). Prior to the t -tests, homogeneity of variances was confirmed with Levene’s test. All statistical analyses were performed in SPSS (SPSS Inc., Chicago, IL, USA). In additional to traditional frequentist statistics, we calculated Bayes Factors ( Supplementary Note 1 ). How to cite this article: Song, S. et al. Practice and sleep form different aspects of skill. Nat. Commun. 5:3407 doi: 10.1038/ncomms4407 (2014).